Inefficient microbial production of refractory dissolved organic matter in the ocean Dissolved organic matter (DOM) in the oceans constitutes a major carbon pool involved in global biogeochemical cycles. More than 96% of the marine DOM resists microbial degradation for thousands of years. The composition of this refractory DOM (RDOM) exhibits a molecular signature ubiquitously detected in the deep oceans. Surprisingly efficient microbial transformation of labile into stable forms of DOM has been shown previously, implying that microorganisms apparently produce far more RDOM than needed to sustain the global pool. Here we show, by assessing the microbial formation and transformation of DOM in unprecedented molecular detail for 3 years, that most of the microbial DOM is different from RDOM in the ocean. Only <0.4% of the net community production is channelled into a form of DOM that is undistinguishable from oceanic RDOM. Our study provides a molecular background for global models on the production, turnover and accumulation of marine DOM. A valuable concept in marine biogeochemistry is the operational definition of dissolved organic matter (DOM) reactivity fractions [1] . Labile DOM comprises organic compounds with lifetimes from minutes to days that mostly escape analysis, while semi-labile and semi-refractory DOM are turned over within 1 to 20 years and accumulate only above a seasonal or permanent pycnocline, respectively. Refractory DOM (RDOM) is the most ubiquitous fraction and resides in the world’s oceans for as long as tens of thousands of years [1] , [2] . RDOM may be formed through abiotic processes, including condensation reactions of low molecular weight DOM [3] , binding of monomers such as amino acids to DOM [4] , microcolloid formation [5] , [6] or exposure to ultraviolet irradiance [4] , [7] . The conceptual framework of the microbial carbon pump [8] summarizes the not yet fully understood biological processes leading to RDOM formation. The microbial transformation of simple substrates produces DOM that persists further degradation for months to years, as demonstrated based on bulk parameters and concentrations of selected compound classes like amino acids and carbohydrates [9] , [10] , [11] , [12] , [13] , [14] . However, <5% of oceanic RDOM consists of these molecularly defined compound classes [15] . An inherent property of RDOM is its enormous molecular diversity that can only be resolved through ultra-high-resolution analytical techniques. One of the most promising techniques is, albeit its limitations, Fourier-transform ion cyclotron resonance mass spectrometry (FT–ICR–MS) [16] . The molecular diversity of microbially formed DOM assessed by this approach is very similar to natural oceanic RDOM [17] , [18] . A currently unresolved conundrum is the observation that RDOM is apparently produced by microorganisms from labile substrates with far higher efficiency than required to sustain the characteristics of the natural DOM pool [11] , [12] , [17] . Hence, the oceanic DOM pool, especially the refractory portion, would be several times larger if the experimentally derived production rates were representative [17] . This obvious paradox with respect to RDOM formation is of concern considering the fact that minor changes in the global RDOM pool could substantially influence atmospheric carbon dioxide concentration and the radiation balance on Earth [8] , [19] . A major caveat of all laboratory experiments is their short duration, compared with the proposed millennium-scale stability [20] of oceanic RDOM. The question remains whether the ‘refractory’ DOM detected in experimental studies is truly equal to oceanic RDOM, having thus the potential to be preserved for thousands of years. To overcome this issue, we here characterize RDOM not only by its stability on an experimental timescale (years), but also by its molecular composition. We define microbially produced RDOM as equal in molecular composition to oceanic RDOM in terms of relative abundance of individual DOM constituents. In contrast, we propose the term ‘pseudo-RDOM’ for the fraction of DOM that survives multiple years of microbial decomposition, but that does not fully match oceanic RDOM in its molecular composition. For this assessment, we combined conventional molecular analysis specifically targeting amino acids and carbohydrates with non-targeted ultra-high-resolution FT–ICR–MS. Thousands of molecular formulae were identified in DOM via this technique [16] , [21] , and further fragmentation studies provided detailed structural information beyond this level [22] . Our results indicate that RDOM, as found in the deep ocean, is generated by diverse microbial communities, but at much lower efficiency than previously assumed based on experimental approaches. DOM production and transformation by microorganisms We inoculated artificial seawater that contained all essential inorganic nutrients but very low background concentrations of dissolved organic carbon (DOC) with a coastal North Sea phytoplankton and bacterial community. This approach was chosen to include as many of the naturally occurring interactions between primary producers and heterotrophic microbes as possible. Over the duration of the experiment (1,011 days), algal and bacterial abundance and community composition, bulk DOC concentration and the molecular composition of solid-phase extracted DOM were monitored. After 167 days, a portion of each mesocosm was filtered and further incubated in the dark (M1–M3 dark ). Three consecutive phases over the course of the mesocosm experiment were identified—the phytoplankton blooms (I), the post-bloom stage (II) and the net-heterotrophic phase (III) of DOM consumption. Between days 1 and 56, favourable experimental conditions ( T ∼ 20 °C, light 120 μmol m −2 s −1 ) with high nutrient supply resembling conditions in upwelling regions or coastal seas [23] induced a sequence of phytoplankton blooms (phase I): the first one was dominated by diatoms ( Thalassiosira minima , Rhizosolenia setigera , Asterionellopsis glacialis ), followed by two smaller blooms with high proportions of flagellates and prymnesiophytes with maxima at days 21 and 38, similar to the natural phytoplankton succession [24] ( Fig. 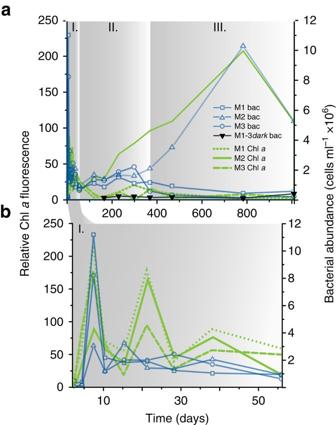Figure 1: Phytoplankton blooms and microbial abundance. (a) Relative chlorophyllafluorescence (M1–M3 Chla) and microbial abundance of the light (M1–M3 bac) and dark (M1–3darkbac: mean microbial abundance of triplicates, s.d. within size of triangles) mesocosms over the course of the experiment and (b) close up of the three phytoplankton blooms until day 56. Roman numerals denote the succession of (I) bloom phase, (II) post-bloom transition and (III) net-heterotrophic phase in the mesocosm microbial community development. 1 , Supplementary Table 1 ). Nitrate and ammonium were depleted below the detection limit within 1 week, while phosphate was never limiting. Bacteria developed diverse communities at densities of 0.2–1 × 10 7 cells ml −1 (free-living fraction Fig. 1 ) that strongly varied among the mesocosms in abundance as well as in composition. The composition of the microbial community was assessed via denaturing gradient gel electrophoresis (DGGE) and the banding patterns subjected to multivariate analysis for graphical representation of sample dissimilarity. Principal coordinates 1 and 2 only explain 19 and 13% of the variation of the microbial community, respectively ( Fig. 2a ), and the samples until day 56 are spread out over the ordination space at an average Bray–Curtis dissimilarity [25] of 0.64±0.1 ( Supplementary Fig. 1b ). 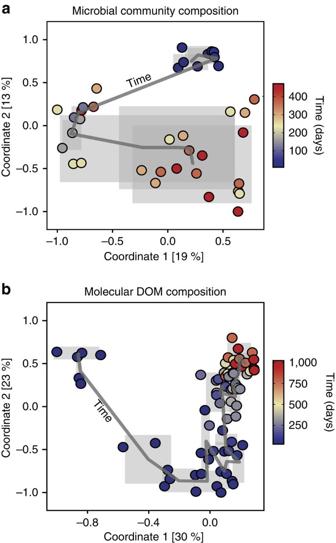Figure 2: Divergence of microbial community composition and convergence of molecular DOM composition. Principal coordinates analysis based on Bray–Curtis dissimilarity of the DGGE-based microbial community composition (a) and the molecular DOM composition (b), colour-coded by time (note the different timescales). The explained variance is given for each of the coordinates 1 and 2. Grey lines average scores at sampling points and illustrate chronological sequence; grey boxes show the s.d. at each sampling point. Members of the Rhodobacteraceae family and some Bacteroidetes representatives were abundant ( Supplementary Table 2 ). About 100 μmol DOC l −1 were generated during the bloom phase regardless of phytoplankton community composition ( Fig. 3 ). The proportion of DOC derived from the total hydrolysable amino-acid concentration (%AA-DOC) peaked during the first phytoplankton bloom with up to 10.5% ( Supplementary Fig. 2i ), indicating freshly produced labile DOM [15] . Also the relative proportion of individual amino acids was consistent with fresh DOM according to the calculated degradation state index [26] ( Supplementary Fig. 2k ). Molecular analysis of solid-phase extracted DOM [27] by FT–ICR–MS revealed that the number of resolved molecular formulae rapidly increased during the first days of the incubation to levels of oceanic RDOM (5800 detected formulae in Pacific water, Supplementary Fig. 2o ). Notably, an increasing proportion (up to 50%) of the newly produced molecular formulae was identical to those found in the Pacific water ( Supplementary Fig. 2t ). 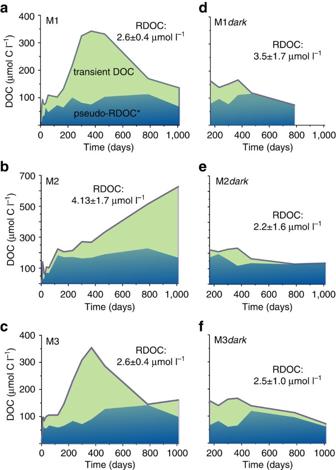Figure 3: DOM fractions according to chemical composition. DOC concentration and contributions of pseudo-RDOC (blue) and transient DOC (green) in light (a–c, M1–M3) and dark (d–f, M1–M3dark) mesocosms. RDOC concentration was averaged for samples taken after day 56. *The calculation of the DOC fractions (transient DOC, pseudo-RDOC, RDOC) was performed for each mesocosm and is described inTable 1. Taking a more detailed look at the mass range of 280–320 Da, where the signal intensities of the mesocosm DOM were highest, as much as 97% of the oceanic molecular formulae were found ( Supplementary Table 3 ). We repeated the FT–ICR–MS analysis in time-consuming, high-sensitivity mode for the mass window of 380–420 Da (where Pacific water had its intensity maximum), and found an 82% agreement of molecular formulae between oceanic and experimental DOM. This finding indicates that a part of the sample similarity is obscured by the detection limit of the FT–ICR–MS, inherent to any analytical method. On the basis of the presence of molecular formulae, the experimental DOM was almost undistinguishable from oceanic RDOM within <2 months of incubation. This is most remarkable, because among the almost 8,000 molecular formulae identified (with the same instrumentation) in the exometabolome of a marine bacterium, a Pseudovibrio strain in monoculture, <2% were identical to DOM from the Pacific water reference sample [28] . We attribute the high number of deep-sea molecular formulae in our experiment to the high microbial diversity and the multitude of possible interactions in the mesocosms. Figure 1: Phytoplankton blooms and microbial abundance. ( a ) Relative chlorophyll a fluorescence (M1–M3 Chl a ) and microbial abundance of the light (M1–M3 bac) and dark (M1–3 dark bac: mean microbial abundance of triplicates, s.d. within size of triangles) mesocosms over the course of the experiment and ( b ) close up of the three phytoplankton blooms until day 56. Roman numerals denote the succession of (I) bloom phase, (II) post-bloom transition and (III) net-heterotrophic phase in the mesocosm microbial community development. Full size image Figure 2: Divergence of microbial community composition and convergence of molecular DOM composition. Principal coordinates analysis based on Bray–Curtis dissimilarity of the DGGE-based microbial community composition ( a ) and the molecular DOM composition ( b ), colour-coded by time (note the different timescales). The explained variance is given for each of the coordinates 1 and 2. Grey lines average scores at sampling points and illustrate chronological sequence; grey boxes show the s.d. at each sampling point. Full size image Figure 3: DOM fractions according to chemical composition. DOC concentration and contributions of pseudo-RDOC (blue) and transient DOC (green) in light ( a – c , M1–M3) and dark ( d – f , M1–M3 dark ) mesocosms. RDOC concentration was averaged for samples taken after day 56. *The calculation of the DOC fractions (transient DOC, pseudo-RDOC, RDOC) was performed for each mesocosm and is described in Table 1 . Full size image After day 56, low chlorophyll a fluorescence prevailed in mesocosms M1 and M3, indicating the post-bloom transition phase (II). In M2, a constant increase in fluorescence until day 785 can most likely be attributed to N 2 -fixing microorganisms in that particular mesocosm. The amino-acid content of the DOC fell below 3% in all light and dark mesocosms similar to the deep ocean and remained low until day 1,011; also the amino-acid degradation state was consistent with oceanic RDOM ( Supplementary Fig. 2k ). Between days 167 and 370, most algal and many bacterial cells lysed, which, together with recycled primary production, resulted in DOC concentrations of up to 350 μmol C l −1 in the light mesocosms ( Fig. 3 ). The dark mesocosms that were started at day 167 showed only little DOC production, presumably derived from decaying cells. From day 370, consumption processes prevailed over new DOM production (net-heterotrophic phase III): bacterial numbers remained low and DOC concentrations decreased by ∼ 200 μmol C l −1 in M1 and M3, but increased by 360 μmol C l −1 in M2 (likely due to continuous N 2 fixation). In all dark mesocosms M1–M3 dark , DOC concentrations decreased by ∼ 90 μmol C l −1 . Despite a strong quantitative variability in DOC concentrations and diverging microbial communities ( Fig. 2a ), molecular DOM composition varied very little over time and among the mesocosms ( Fig. 2b ). The narrow range of molecular composition, for example, of average H/C (1.37±0.02) and O/C (0.40±0.01) ratios of the dissolved molecules after day 300, is mirrored by the low Bray–Curtis dissimilarity of the DOM of 0.27±0.16 ( Fig. 1 , Supplementary Fig. 2r,s ). The diverse phytoplankton and bacterial community in our batch incubations produced molecularly highly diverse DOM with an apparently enormous similarity to oceanic RDOM. After initial injection of 40 μmol inorganic nitrogen l −1 (as the limiting element) newly produced DOM in the copious amount of ∼ 100 μmol DOC l −1 remained after 3 years. This production efficiency of apparent RDOM largely exceeds—by more than one order of magnitude—the efficiency needed to sustain the global RDOM inventory [1] . In this sense, our study is consistent with the above mentioned conundrum revealed by previous studies [11] , [12] , [17] . If, however, the molecular similarity with oceanic RDOM is extended towards the level of molecular structures and especially abundance patterns, a very different picture emerges. One molecular formula may represent a multitude of structural isomers. To reveal structural features behind the molecular formulae, we fragmented in the FT–ICR–MS a total of 32 abundant formulae of six masses belonging to two homologous series of Pacific water and a pooled M3 sample ( Fig. 4 ). The applied fragmentation approach is not aiming at unambiguous structure determination, but it provides information about the overall presence and relative frequency of molecular building blocks behind a given molecular formula. Thus, the fragmentation patterns are structural fingerprints that aid in the decision whether different structural isomers hide behind a given molecular formula of different samples. The major fragmentation patterns revealed the prevalence of organic acids in both samples (that is, combinations of CO 2 , H 2 O and CH 4 O fragments). Other structural features such as esters, ethers or peptides were rare in both samples. Despite this overall structural similarity, the abundance patterns of the respective fragments were different ( Fig. 4 ), indicating that the structural composition of oceanic RDOM and DOM produced in the mesocosms was not identical. 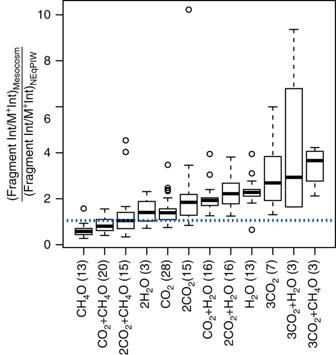Figure 4: Structural dissimilarity revealed by fragmentation. FT–ICR–MS collision fragmentation was conducted for six nominal masses (32 molecular formulae) contained in Pacific and mesocosm DOM. The fragmentation patterns describe the molecular dissimilarity on a structural level. The boxplot depicts the ratios of the relative fragment intensities (relative to the respective parent ion) of mesocosm and Pacific DOM (NEqPIW), grouped by the type of neutral loss. Only fragments occurring in both samples were considered. The same structures behind a molecular formula would yield a ratio of 1 (dotted blue line). The number behind each neutral loss formula denotes the number of molecular formulae for which the respective loss was detected. Figure 4: Structural dissimilarity revealed by fragmentation. FT–ICR–MS collision fragmentation was conducted for six nominal masses (32 molecular formulae) contained in Pacific and mesocosm DOM. The fragmentation patterns describe the molecular dissimilarity on a structural level. The boxplot depicts the ratios of the relative fragment intensities (relative to the respective parent ion) of mesocosm and Pacific DOM (NEqPIW), grouped by the type of neutral loss. Only fragments occurring in both samples were considered. The same structures behind a molecular formula would yield a ratio of 1 (dotted blue line). The number behind each neutral loss formula denotes the number of molecular formulae for which the respective loss was detected. Full size image On the basis of general chemical properties and molecular characteristics, we defined three fractions of microbially produced DOM ( Table 1 , Fig. 3 ). The ‘transient DOM’ constituted the fraction most dissimilar to oceanic RDOM and was also most dynamic. It slowly accumulated but was then nearly completely degraded in the net-heterotrophic phase. The high C/N ratio ( Supplementary Fig. 2c ) of the molecules was consistent with a high contribution of dissolved combined carbohydrates to the remaining pseudo-RDOM at day 1,011 (M1, M3 ∼ 3 μmol l −1 , M2 ∼ 26 μmol l −1 , M1–M3 dark <1 μmol l −1 ). We defined ‘pseudo-RDOM’ as being very similar but not fully identical to oceanic RDOM, both with respect to bulk chemical properties and molecular characteristics. Pseudo-RDOM was formed during the bloom phase and remained at concentrations of ∼ 100 μmol C l −1 . We propose that much of the DOM in this class had previously been termed RDOM because of its longevity on experimental timescales and chemical similarity to oceanic RDOM. Ultra-high-resolution mass spectrometry enabled us to define the smallest experimental DOM fraction: it is equal to oceanic RDOM in terms of presence and relative intensities of resolved masses. To match this definition, the molecular formulae detected in oceanic RDOM cannot be larger in relative intensity to their respective counterparts in the mesocosm DOM sample on a given confidence level of 99%. On the basis of this definition, at most 2.9±1.4 μmol C l −1 of RDOM existed in the mesocosm DOM at day 56 and thereafter, representing <0.18–0.36% of the net community production in the mesocosms (NCP; new production based on inorganic nitrogen and phosphate uptake). For this estimate, we assume that all molecular formulae that are shared between oceanic RDOM and mesocosm DOM consist of the same structural isomers, while at the same time we show through the fragmentation experiments that this is not the case. Therefore, our calculation conservatively overestimates, but by no means underestimates the production of RDOM. Especially in light of this possible overestimation, it is remarkable that our experimentally derived biogenic RDOM production rates (0.18–0.36% of NCP) are in the same order of magnitude as the estimates derived from global DOC distribution patterns (0.63% of NCP) [1] , [29] . Also the observed production of ‘pseudo-RDOM’ is consistent with estimates on the total oceanic production of semi-labile and semi-RDOM [1] , [29] . Table 1 Reactivity of DOM fractions. Full size table Photochemical alteration [30] , thermogenic processes [31] and other abiotic factors may contribute to the formation of RDOM, but our study indicates that diverse microbial communities alone produce DOM that is similar in reactivity and composition to RDOM found in the global ocean. We were able to shed light and provide experimentally derived data on the production of large amounts of seemingly RDOM in mesocosm experiments and conclude that less RDOM than previously thought [8] , but still enough to sustain the global RDOM pool, is produced by microorganisms. The underlying mechanisms behind the relationship between NCP and RDOM production remain to be understood, particularly in consideration of the yet unknown implications of global change [19] , [32] on DOM dynamics. Experimental set-up At the start of the mesocosm experiment, 9.9 l artificial seawater (Difco Marine Broth 2216 (ref. 33 ) without yeast extract and peptone, DOC 7.4 μmol C l −1 ) were transferred into acid-rinsed 10 l glass bottles and mixed with 0.1 l of prefiltered (200 μm) coastal North Sea water (Norderney, Germany, 30 May 2011, 53°31’48’N 7°9’26’E, DOC 247 μmol l −1 ) in triplicates (M1, M2, M3). The mesocosms were incubated at room temperature (average 22.5 °C), 12:12 hour light:dark (120 μmol m −2 s −1 , 400–700 nm) and the water was constantly stirred. After 167 days, 1.5 l of each mesocosm were filtered through 1.2-μm glass fibre filters (Whatman, precombusted 400 °C, 4 h) to remove aggregates and phytoplankton, and then further incubated in the dark (M1 dark , M2 dark , M3 dark ). At each of the 17 sampling points, 300–400 ml were withdrawn from the 10 l bottles and further processed and preserved for the analyses. A control consisted of the same set-up, but contained ultrapure water. Phytoplankton and chlorophyll a Relative chlorophyll a fluorescence was determined fluorometrically at every sampling point (excitation 540 nm, emission 684 nm, TD-700 Fluorometer, Turner Designs, USA). Enumeration and classification of phytoplankton was performed at five time points during the experiment in triplicates by AquaEcology (Oldenburg, Germany, Supplementary Table 1 ). Additional confirmation of the presence of cyanobacteria that were not identified by direct counts was obtained via flow cytometric investigation of the autofluorescence of live samples on day 473. High phycobilin fluorescence provides strong evidence for a population of Synechococcus sp. (1.6 × 10 5 cells ml −1 ) in M2 and of Prochlorococcus sp. (4.4 × 10 3 cells ml −1 ) in M1 (ref. 34 ). M3 did not exhibit phycobilin fluorescence on day 473. Microbial cell counts and community analysis The determination of cell numbers of the free-living microorganisms was conducted with a BD Accuri C6 cytometer (BD Biosciences, USA) using SybrGreen I (Invitrogen, United Kingdom) after staining and the internal fluidics calibration of the device. The fixed samples (2% final concentration glutardialdehyde, Carl Roth, Germany) were filtered through 50 μm filters (Cell Trics, Partec) to remove larger particles. Volume verification was done using TruCount beads (BD) as described previously [35] , [36] . For the analysis of the bacterial community composition by DGGE [37] of PCR-amplified 16S rRNA gene fragments, 30–40 ml of the sample were passed through 0.2 μm polycarbonate filters (Millipore, USA). DNA extraction and DGGE was conducted as described in Osterholz et al. [21] . The DNA of prominent, excised bands was reamplified and purified (Gold DNA purification kit, Quiagen, Netherlands) before sequencing at GATC Biotech AG (Germany). The obtained sequences were compared with those in GenBank using the Blast tool ( www.ncbi.nlm.nih.gov ) and results are summarized in Supplementary Table 2 . Quantification of inorganic nutrients Subsamples for nutrient analysis (NH 4 + , NO 3 − , NO 2 − , PO 4 3− , Supplementary Fig. 2d–g ) were filtered (0.2 μm, Isopore Membrane Filter, EMD Millipore Corporation, USA) and preserved with HgCl 2 . PO 4 3− and NH 4 + were analysed via micro-photometric methods [38] . NO 3 − and NO 2 − were determined via vanadium(III)chloride reduction [39] . Amino-acid quantification Aliquots for the quantification of total dissolved hydrolysable amino acids (THDAA) were filtered (0.2 μm, Acrodisc, PALL Life Science, USA) and quantified after orthophthaldialdehyde precolumn derivatization as described in Lunau et al. [40] on a high-performance liquid chromatography system (HPLC, 1200 series, Zorbax Eclipse XDB-C18-4.6 × 12.5 mm precolumn, Zorbax Eclipse XDB-C18-4.6 × 150 mm main column, Agilent Technologies, USA). Aspartic acid, glutamic acid, histidine, serine, arginine, glycine, threonine, alanine, tyrosine, methionine, valine and phenylalanine were resolved and quantified via external standards ( Supplementary Fig. 2h–j ). The degradation state index DI ( Supplementary Fig. 2k ) was calculated after Dauwe et al. [26] . Carbohydrate quantification Samples for dissolved total neutral carbohydrates (DCCHO) were prepared in the same way as for THDAA quantification, but only analysed in the sample of day 1011. DCCHO (glucose, mannose, galactose, fucose, rhamnose, arabinose, xylose) quantification was performed by HPLC with a Carbopac PA 1 column (Dionex, Thermo Fisher Scientific Inc., USA) and pulsed amperometric detection [41] . DOC and TDN quantification The sample was filtered (0.2 μm Isopore Membrane Filter, EMD Millipore Corporation, USA) and acidified to pH 2 (HCl 25% p.a., Carl Roth, Germany). Duplicate quantification of DOC ( Supplementary Fig. 2a ) and total dissolved nitrogen (TDN, Supplementary Fig. 2b ) was performed via high-temperature catalytic combustion using a Shimadzu TOC-VCPH/CPN Total Organic Carbon Analyzer equipped with an ASI-V autosampler and a TNM-1 module [21] . For the calculation of molar C/N ratios of DOM, the inorganic nitrogen concentration was subtracted from TDN ( Supplementary Fig. 2c ). The accuracy of DOC and TDN quantification was confirmed by analysing deep-sea reference samples provided by the University of Miami (Dennis Hansell). The error of DOC and TDN analysis was on average 4 and 10%, respectively. The DOC concentration in a control treatment (consisting of ultrapure water only) never exceeded 12.3 μmol l −1 over the course of the experiment. Solid-phase extraction and FT–ICR–MS analysis DOM was solid-phase extracted from filtered and acidified samples (150–250 ml) with commercially available PPL columns (100 mg, Agilent, USA) [27] . After extraction, cartridges were rinsed with acidified ultrapure water (pH 2, HCl 25%, p.a., Carl Roth, Germany), dried with argon gas and eluted with 500 μl of methanol (HPLC-grade, Sigma-Aldrich, USA). The extraction efficiency increased during the experiment from 9.9% to up to 69.3% (average: 35.1±14.2%) on a carbon basis. The concentration of extractable DOC was determined in the solid-phase extracts after complete removal of the methanol and dissolution in ultrapure water ( Supplementary Fig. 2m,n ). The mass spectra were obtained on a 15 T Solarix FT–ICR–MS (Bruker Daltonics, USA) equipped with an electrospray ionization source (Bruker Apollo II) applied in negative mode. DOM extracts from day 4 on were diluted to a final DOC concentration of 20 mg C l −1 in a 1:1 (v/v) mixture of ultrapure water and methanol (HPLC-grade, Sigma-Aldrich, USA). For routine analyses, 500 scans were accumulated per run in a mass window from 150 to 2,000 Da. The spectra were mass calibrated with an internal calibration list using the Bruker Daltonics Data Analysis software package and processed using in-house Matlab routines. Diluted octaethylene glycol solution (PEG-8, H(OCH 2 CH2) 8 -OH, ≥95% oligomer purity, Sigma-Aldrich) was added to the diluted extracts as an internal standard before FT–ICR–MS analysis for better quantitative comparison of the spectra. Molecular formulae were assigned to masses with a minimum signal-to-noise ratio of 4 following the rules published in Koch et al. [42] . The number of assigned molecular formulae, average intensity-weighted molecular masses, double bond equivalents (DBE), H/C ratios and O/C ratios ( Supplementary Fig. 2o–s ) were calculated for each sample. Reference samples The North Sea inoculum was solid-phase extracted as described above and analysed repeatedly via FT–ICR–MS ( n =15) to provide an estimate of the background DOM introduced into the mesocosms at the start. The oceanic RDOM reference sample was North Equatorial Pacific Intermediate Water (NEqPIW [43] ) obtained from 674 m depth near Hawaii in the oxygen minimum zone (20–30 μM O 2 ) [44] using the same extraction method [45] . The NEqPIW ranges among the older water masses on earth [43] , [46] and can thus be considered to carry primarily RDOM [1] . The reference sample was measured repeatedly ( n =12) to assess possible instrument variability and used for comparison with the spectra of the incubated DOM. DOM fragmentation experiments To explore the structural agreement between assigned molecular formulae detected in the NEqPIW reference sample and the mesocosms, we fragmented three nominal masses of two CH 2 -homologous series (32 molecular formulae), respectively, in the NEqPIW reference and a pooled mesocosm sample (M3, days 370, 469, 785). The nominal masses (269, 283, 297, 327, 341 and 365 Da) were isolated in the quadrupole unit of the FT–ICR–MS and fragmented in a hexapole unit via collision with argon. The collision energy was optimized for each mass, but kept the same between the two samples. Samples were run in negative mode using ESI ionization, injected at 100 mg C l −1 , and 150 broadband scans were accumulated per run. Fragmentations were conducted in triplicate for each nominal mass. A total of 267 different fragments were identified, resulting from the neutral loss of the following 12 units—H 2 O, CH 4 O, 2H 2 O, CO 2 , CO 2 +H 2 O, CO 2 +CH 4 O, 2CO 2 , 2CO 2 +H 2 O, 2CO 2 +CH 4 O, 3CO 2 , 3CO 2 +H 2 O and 3CO 2 +CH 4 O. All 12 neutral losses were observed in both samples. Only molecular formulae that were detected in all three replicate measurements were considered for data evaluation. Of the 267 identified fragments, 152 (57%) were found in both samples. Results from these common fragments are shown in Fig. 4 . Of the 115 fragments that were only detected in one of the samples, 84 were present only in the mesocosm DOM and 31 were present only in the NEqPIW. For mother ions of low intensity, fragments may be below detection limit. Considering the signal intensity ratio of mother to daughter ion and the detection limits of FT–ICR–MS, of the 84 exclusive mesocosm DOM fragments, 49 possible fragments may have been below the detection limit in the NEqPIW sample, while 35 fragments should have been detectable. All of the exclusive NEqPIW DOM fragments should have been above detection limit in the mesocosm DOM. To fully eliminate possible artifacts introduced by the detection limit, we restrict the discussion only to those fragments that were reliably detectable in both samples. Estimate of RDOM concentration The approach used to estimate RDOM concentrations assumes a linear response signal of the FT–ICR–MS, that is, a linear increase of the signal in response to increasing concentration of the respective compounds. This was experimentally confirmed by injecting the NEqPIW DOM at different concentrations from 4 to 20 mg C l −1 amended with the polyethylene glycol internal standard as described above ( Supplementary Fig. 3 ). Furthermore, it was assumed that the same compounds have the same response signal if analysed in the sample matrix of NEqPIW and the mescosom. We tested for possible matrix effects by mixing NEqPIW with the pooled mesocosm sample (M3, days 370, 469, 785) in 10% increments. The resulting 7 samples (0/100, 10/90, ..., 50/50, 100/0% of NEqPIW/mesocosm, data not shown) were analysed on the FT–ICR–MS. The actual measured signal intensities of each detected mass were compared with the mathematically predicted intensity that results from the linear mixing ratios of the endmembers. There was no detectable difference between measured and calculated peak intensities ( P <0.0001). A matrix effect was therefore excluded for our study. Estimate of RDOM concentration We define ‘true’ RDOM as equal in molecular composition to abyssal RDOM in terms of relative abundance of individual DOM molecular formulae. Masses with assigned molecular formulae that were detected in all 12 independent FT–ICR–MS analyses of NEqPIW DOM, which is here defined as ‘true RDOM’, were taken into account for the estimation of RDOM concentration in the mesocosm DOM. The sum of the considered signal intensities was not statistically different between the NEqPIW and the mesocosm DOM before normalization (Mann–Whitney U -test, two-tailed, P >0.3), that is, the response signal of the FT–ICR–MS was independent of the type of sample in our experiment. Before sample comparison, each sample was normalized to its sum of signal intensities. Then, the average intensity of each NEqPIW molecular formula (NEqPIW I ) from which the standard deviation of all NEqPIW analyses ( n =12) multiplied by σ =2.576 (99% confidence level) had been subtracted to conservatively account for analytical variability was divided by the intensity of the respective mesocosm molecular formula (MC I ) ( Supplementary Fig. 4 ). Each intensity ratio (NEqPIW I /MC I ) was then log-transformed to obtain normal distribution. The number of outliers was determined by counting the log-transformed ratios that deviated from the normal distribution by more than 2.576 times the s.d. per sample (99% confidence level). This confidence level was chosen because it allowed us to fit at least 100% of each NEqPIW mass spectrum into the average NEqPIW spectrum used also for comparison with the mesocosm DOM. By means of this method, on average, 33 molecular formulae per sample ( ∼ 0.3% of all formulae) were excluded from the fit. The resulting highest (NEqPIW I /MC I ) max signal intensity ratio determined the percentage of NEqPIW DOM that can be fitted into the mesocosm DOM ( Supplementary Fig. 4 ), after consideration of the confidence level and removal of outliers: In other words, the molecular formula that had the lowest intensity in the mesocosm compared with its counterpart in NEqPIW is the limiting factor in this fit. At last, this percentage was multiplied by the solid-phase extractable DOC concentration (μmol C l −1 ) and a factor of 3/2 to account for the solid-phase extractability of RDOM ( ∼ 2/3 for NEqPIW [45] ) to derive the respective RDOC concentration contained within the mesocosm DOC. This concentration was then used to calculate the percentage of the NCP of DOC transformed into RDOC. NCP and global estimates The NCP constitutes the difference between gross primary production and total respiration of a community. We assumed a ratio of carbon to nitrogen uptake at Redfield stoichiometry [29] (C:N:P = 106:16:1 (ref. 47 )) and estimated the NCP from the uptake of inorganic nitrogen (nitrate and ammonium) or phosphate during the phase of new production until day 56 in our mesocosms: The nitrogen-based new production was on average (M1, M2 and M3) 286±5 μmol C l −1 through the uptake of 43.1±0.8 μmol l −1 inorganic nitrogen in form of nitrate and ammonium. Since nitrogen fixation cannot be ruled out in our mesocosms, we additionally calculated the phosphorus-based new production: 4.1±0.7 μmol P l −1 were assimilated, resulting in a new production of 439±77 μmol C L −1 . It has to be noted that the biological drawdown of inorganic carbon and nitrogen was underestimated in some oceanic regions [48] when a Redfield stoichiometry was assumed, but we regard the accuracy as sufficient for the purposes of this study. Among others, one important motivation for the implementation of this study was the fact that previous studies have reported RDOM production rates that exceeded the amounts needed to sustain the global RDOM pool by far ( Supplementary Table 4 ). According to the results presented in this study, a maximum of 0.2–0.4% of the NCP of the mesocosms were channelled into the RDOM pool. This result is within the order of magnitude of the estimated global RDOM production from NCP of 0.6% (ref. 29 ). Multivariate statistics DGGE banding patterns were translated into a numerical table and normalized before analysis. Relative FT–ICR–MS signal intensities were also normalized to the sum of intensities per sample; only masses with assigned molecular formulae were used. Bray–Curtis [25] , [49] dissimilarity matrices ( Supplementary Fig. 1 ) were constructed for both data sets, and PCoA (principal coordinates analysis, Fig. 2 ) was chosen for graphical representation of the variability of samples over time based on the two major axes of variation. The analyses were performed in R (version 3.1.1, R Development Core 'Team 2012, [ http://cran.r-project.org/ ]) and using the package ‘vegan’ [50] . Accession codes : Sequences are deposited at GenBank under accession number KJ914554 to KJ914571 . All data are available via the PANGAEA data library (doi:10.1594/PANGAEA.840595). How to cite this article: Osterholz, H. et al. Inefficient microbial production of refractory dissolved organic matter in the ocean. Nat. Commun. 6:7422 doi: 10.1038/ncomms8422 (2015).